Motion-based DNA detection using catalytic nanomotors Synthetic nanomotors, which convert chemical energy into autonomous motion, hold considerable promise for diverse applications. In this paper, we show the use of synthetic nanomotors for detecting DNA and bacterial ribosomal RNA in a fast, simple and sensitive manner. The new motion-driven DNA-sensing concept relies on measuring changes in the speed of unmodified catalytic nanomotors induced by the dissolution of silver nanoparticle tags captured in a sandwich DNA hybridization assay. The concentration-dependent distance signals are visualized using optical microscopy, particularly through straight-line traces by magnetically aligned 'racing' nanomotors. This nanomotor biodetection strategy could be extended to monitor a wide range of biomolecular interactions using different motion transduction schemes, thus providing a versatile and powerful tool for detecting biological targets. Wide-scale genetic testing requires the development of easy-to-use, fast, inexpensive, miniaturized analytical devices. DNA hybridization biosensors commonly rely on different types of optical [1] , [2] , electrochemical [3] , [4] and mechanical [5] transducers to convert duplex formation recognition events into useful analytical signals. Nanomaterial tags have greatly benefited such bioassays through amplified or multiplexed measurements [6] , [7] . However, autonomously propelling nanoscale materials have not been exploited for biosensing applications. Chemically powered nanomotors, particularly bisegment Au–Pt nanowires, exhibit autonomous propulsion because of the electrocatalytic decomposition of hydrogen peroxide fuel [8] , [9] , [10] , [11] , [12] . Previous efforts in the field of synthetic nanomotors have concentrated on increasing their speed and power and in imparting precise motion control and cargo-towing capabilities. Factors influencing the nanomotor speed, including motor and fuel compositions, along with new motor capabilities, have been reviewed elsewhere [8] , [9] , [10] . Recently, we discovered an unusual increase in the speed of catalytic nanowire motors in the presence of silver ions [13] . In this paper, we present a fundamentally new nanomotor-based biodetection platform for specific DNA and RNA detection. Silver-induced nanomotor speed enhancement is used in a sensitive, rapid and simple hybridization assay. Our motion-based hybridization sandwich assay relies on the duplex formation of the nucleic acid target with a thiolated DNA capture probe and a silver nanoparticle-tagged detector probe (SH-DP-Ag NPs). Subsequent dissolution of the Ag nanoparticle tags in the hydrogen peroxide fuel releases Ag ions, which, on adding an aliquot of the unmodified nanomotor solution, causes a substantial increase in their speed. The higher the concentration of the nucleic acid target, the more the silver nanoparticles (Ag NPs) that are captured, and the greater the nanomotor speed. The resulting distance signals allow convenient measurements of the DNA target down to the attomole level. This new nanomotor concept may be readily expanded for detecting protein markers in connection with antibody or aptamer receptors. The motility of motor proteins has been proposed recently for transporting and detecting target biomolecules [14] , [15] . However, there are no reports on using synthetic nanomotors for transducing biorecognition events into motion. Such artificial nanomachines address the limitations of using biological motors, including a limited lifetime in vitro and a narrow functioning range of environmental conditions [16] . 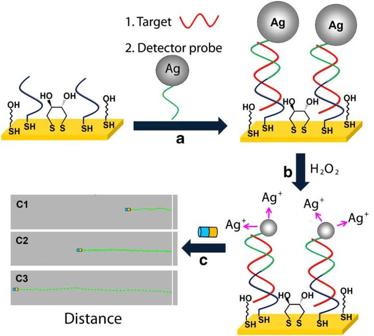Figure 1: Motion-based nucleic acid detection. (a) Hybridization of the target and capture of the Ag nanoparticle-tagged detector probe in a typical sandwich assay on the ternary SH-CP/DTT+MCH surface, including washing of unbound SH-DP-Ag NPs. (b) Dissolution of silver nanoparticle tags in the peroxide fuel, leading to Ag+-enriched fuel. (c) Visual detection of the motion of the catalytic nanowire motors in the resulting Ag+-enriched fuel. C1, C2 and C3 represent hypothetical and increasing target nucleic acid concentrations. Motion-based nucleic acid detection assay The principle behind motion-based nucleic acid detection using catalytic nanomotors is illustrated in Figure 1 . Initially, a gold electrode is modified with a ternary monolayer composed of a thiolated capture probe (SH-CP), mercaptohexanol (MCH) and dithiothreitol (DTT). The presence of a complementary nucleic acid target leads to duplex formation and subsequent capture of a SH-DP-Ag NP. After the washing step to remove the excess unbound SH-DP-Ag NPs, hydrogen peroxide is added, leading to rapid dissolution of the captured nanoparticle tags into silver ions. The Ag + -enriched fuel is separated from the surface of DNA modified gold electrode and directly added to an equal volume of freshly prepared nanomotor solution, thereby leading to a change in their speed and hence to concentration-dependent nanomotor distance signals. Such signals can be easily and directly traced using optical microscopes, hence obviating the need for sophisticated analytical instruments. Figure 1: Motion-based nucleic acid detection. ( a ) Hybridization of the target and capture of the Ag nanoparticle-tagged detector probe in a typical sandwich assay on the ternary SH-CP/DTT+MCH surface, including washing of unbound SH-DP-Ag NPs. ( b ) Dissolution of silver nanoparticle tags in the peroxide fuel, leading to Ag + -enriched fuel. ( c ) Visual detection of the motion of the catalytic nanowire motors in the resulting Ag + -enriched fuel. C1, C2 and C3 represent hypothetical and increasing target nucleic acid concentrations. Full size image Ag NP-induced nanomotor acceleration Silver nanoparticle tags, commonly used in optical [17] or electrochemical [18] DNA detection, are rapidly dissolved in the hydrogen peroxide fuel and the resulting silver ions lead to a dramatic speed increase in nanomotors, in accordance with early observations [13] . 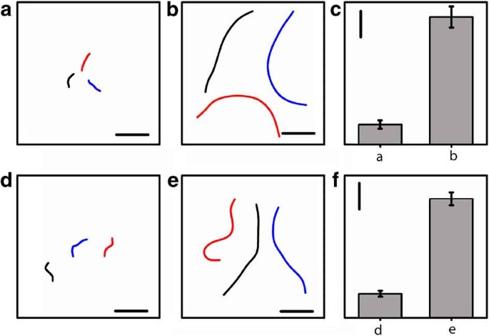Figure 2: Tag-induced nanomotor acceleration. Track lines of nanomotors illustrating the distances travelled by three Au–Pt nanowires over a 1 s period in the presence of 10% H2O2(a) and 10% H2O2containing 40 pM Ag nanoparticles (b). Scale bar, 10 μm. The corresponding column graph is shown inc. Traces of three nanomotors over a 1 s period in the presence of 15% H2O2following complete hybridization assays using 0 nM (d) and 100 nM target DNA (e). The corresponding column graph is shown inf. Error bars estimated as a triple of the standard deviation (n=20). The accelerated motion of catalytic nanomotors in the presence of Ag NPs is illustrated in Figure 2a–c . It compares traces of three Au–Pt nanomotors, taken over a period of 1 s, in the presence of 10% H 2 O 2 fuel without ( Fig. 2a ) and with 40 pM Ag NPs ( Fig. 2b ). The nanowires exposed to nanoparticles travel substantially longer distances compared with those present in the fuel solution not containing nanoparticles (49.2 versus 7.7 μm; Fig. 2c ), thereby reflecting a 6.4-fold speed enhancement. Videos illustrating such increased propulsion of Au–Pt nanomotors in the presence of Ag NPs are displayed in Supplementary Movie 1 . The complete and instantaneous dissolution of Ag NPs in the peroxide fuel was confirmed by UV–Visible spectroscopy ( Supplementary Fig. S1 ). A silver ion concentration of 40 μM was estimated from the number of ions released by a 40 pM silver nanoparticle solution (based on the packing density ratio). The speed increase (to around 50 μm s −1 ) observed for this Ag + concentration correlates well with the expected silver effect [13] . Figure 2: Tag-induced nanomotor acceleration. Track lines of nanomotors illustrating the distances travelled by three Au–Pt nanowires over a 1 s period in the presence of 10% H 2 O 2 ( a ) and 10% H 2 O 2 containing 40 pM Ag nanoparticles ( b ). Scale bar, 10 μm. The corresponding column graph is shown in c . Traces of three nanomotors over a 1 s period in the presence of 15% H 2 O 2 following complete hybridization assays using 0 nM ( d ) and 100 nM target DNA ( e ). The corresponding column graph is shown in f . Error bars estimated as a triple of the standard deviation ( n =20). Full size image Motion-based detection of DNA and Escherichia coli 16S rRNA The instantaneous dissolution of metal nanoparticles in the fuel solution and the resulting silver-induced accelerated motion are the bases for using nanomotors to detect nucleic acid hybridization. Figure 2d–f compares traces of three Au–Pt nanomotors swimming (over a period of 1 s) in the peroxide fuel solution after complete hybridization assays with 0 and 100 nM DNA target ( Fig. 2d, e , respectively). Such results are further demonstrated in Supplementary Movie 2 . The 100 nM DNA target leads to an average travel distance of 45.9 μm ( Fig. 2e ), compared with the 9.2 μm signal observed for the control hybridization experiment without target ( Fig. 2d ). Similar traces recorded for intermediate DNA target concentrations of 10 pM, 100 pM, 1 nM and 10 nM yielded increasing speeds of 11.5, 18.7, 24.9 and 31.5 μm s −1 , respectively. The resulting calibration plot ( Supplementary Fig. S2 ) shows a clear concentration dependence. Straight-line distance signals of 'racing nanomotors', accomplished by incorporating a ferromagnetic nickel segment into the nanowire motors [19] along with a directed magnetic alignment, provide an extremely convenient and attractive quantitation of the DNA targets. 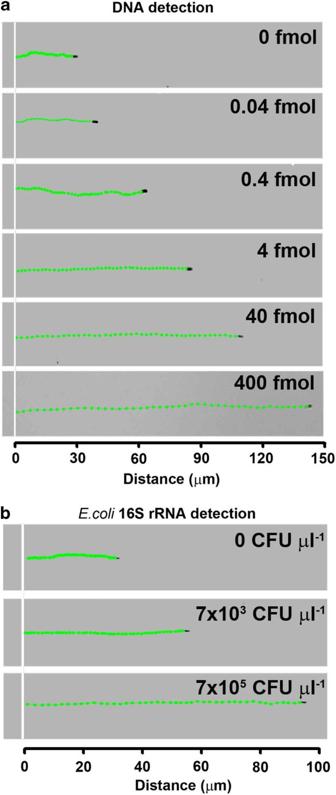Figure 3: Nanomotor racing for quantitative nucleic acid detection. Motion-based DNA detection of different levels of synthetic target (a) and ofE. coli16S rRNA (b) corresponding to different cell concentrations (CFU, colony-forming units). Optical images superimposed with straight-line track lines illustrating the distance travelled by the corresponding Au–Ni–Au–Pt nanomotors over a 4 s period. The optical images of Figure 3a illustrate such straight-line hybridization signals, recorded over a 4 s period, for 4 μl samples containing increasing levels of the DNA target over the 40 amol–400 fmol range (that is, 10 pM–100 nM), along with the control (0 DNA) solution. Such directional motion control allows for a clear visual comparison of the distance readouts of the different DNA concentrations. As expected, longer signals—ranging from 37.2 to 144.0 μm—are observed upon increasing the DNA concentration. A well-defined concentration dependence is therefore obtained over the broad 40 amol–0.4 pmol range ( Fig. 3a and Supplementary Fig. S3a ). Supplementary Movie 3 illustrates the straight-line 'race' of the Au–Ni–Au–Pt nanomotors in connection with the different DNA concentrations, and hence the attractive performance of the new motion biodetection platform. The nanomotor distance signal for the 40 amol DNA solution was shown to be statistically different when compared with a control, with an average speed of 9.3 μm s −1 (versus 7.3 μm s −1 , respectively). This detection limit compares favourably with those reported for other nanostructure-based DNA assays [6] . Such a value is particularly impressive, considering the simplicity of the developed methodology and the absence of any deliberate amplification protocol, such as Ag enhancement or target PCR. Even lower levels of the DNA target could be detected by recording the distance signals over longer time, thereby making small concentration differences more discernable (in a manner reminiscent of increasing the electrophoresis gel running time to distinguish between similarly sized fragments). Figure 3: Nanomotor racing for quantitative nucleic acid detection. Motion-based DNA detection of different levels of synthetic target ( a ) and of E. coli 16S rRNA ( b ) corresponding to different cell concentrations (CFU, colony-forming units). Optical images superimposed with straight-line track lines illustrating the distance travelled by the corresponding Au–Ni–Au–Pt nanomotors over a 4 s period. Full size image The practical utility of this new motion-driven DNA assay was illustrated using the same capture and detector probe for the detection of 16S rRNA which is released from E. coli pathogenic bacteria and obtained from a previously reported sample preparation [20] , [21] . Figure 3b and the corresponding Supplementary Movie 4 show catalytic nanomotors 'racing' following hybridization assays using different bacterial lysate solutions corresponding to different E. coli cell concentrations: 0, 7×10 3 and 7×10 5 CFU μl −1 , leading to average distance signals of 32, 56 and 96 μm, respectively ( Fig. 3b and Supplementary Fig. S3b ). The results indicate a sensitive detection of the genetic material corresponding to around 2,000 E. coli CFU μl −1 level. Specificity and precision studies The specificity of the motion-sensing protocol was examined by challenging the system with excess of various non-complementary and mismatched oligonucleotides. 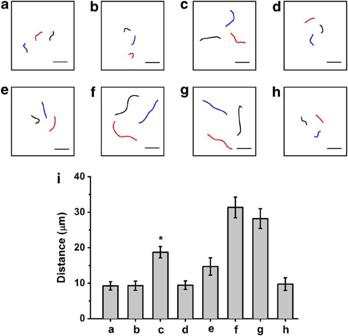Figure 4: Specificity of the motion-driven nucleic acid detection. Track lines illustrating the distances travelled by three nanomotors over a 1 s period in 15% H2O2after hybridization with 0 nM target DNA (normal control) (a), large excess (1 μM) of a non-complementary DNA (b), 100 pM of the DNA target (c), large excess (1 μM) of a three-base mismatched oligonucleotide (d), 10 nM two-base mismatched oligonucleotide (e), 10 nM target DNA (f), 16S rRNA corresponding to 5×105CFU μl−1E. coli(g) and 16S rRNA corresponding to 7×105CFU μl−1K. pneumoniae(h). Scale bar, 10 μm. The corresponding column graph was shown ini. Error bars estimated as a triple of the standard deviation (n=20). *Indicates a significance value ofP<0.001. Figure 4 shows distance signals to 0 (a), 100 pM (c) and 10 nM (f) of target DNA, along with the nanomotor response to a large excess of non-complementary and mismatched oligonucleotides (b, d and e). The corresponding column graph ( Fig. 4i ) provides a quantitative summary of these data. As expected, the system responds favourably to the target DNA with well-defined distance signals of 18.7 and 31.5 μm for the 100 pM and 10 nM levels, respectively. In contrast, a huge excess (1 μM) of non-complementary ( Fig. 4b ) and three-base mismatched ( Fig. 4d ) oligonucleotides displays a negligible change in the response (compared with the control signal without the nucleic acid; Fig. 4a ). Only the two-base mismatched DNA ( Fig. 4e ) yields a defined signal of 14.7 μm (compared with 31.5 μm for a similar level of the complementary DNA target, Fig. 4f ). Such response reflects the partial duplex formation of the mismatch, hence the capture of the Ag NP 'accelerating' tags. Supplementary Movie 5 shows the movement of nanomotors after hybridization assays with 1000 nM non-complementary oligonucleotieds, 0 nM (control experiment) and 100 pM of target DNA. Overall, the data of Figure 4 and Supplementary Movie 5 indicate that the motion detection platform offers high specificity, reflecting the negligible non-specific adsorption of the SH-DP-Ag NPs onto the mixed self-assembled monolayer on the gold surface. The small background contributions compare favourably with those of analogous nanoparticle-based bioassays [17] , [18] . Further discrimination against more closely mismatched oligonucleotides, such as single mismatched DNAs, could be achieved by stringent control of hybridization conditions or by using highly specific peptide nucleic acid capture probes [22] . Figure 4: Specificity of the motion-driven nucleic acid detection. Track lines illustrating the distances travelled by three nanomotors over a 1 s period in 15% H 2 O 2 after hybridization with 0 nM target DNA (normal control) ( a ), large excess (1 μM) of a non-complementary DNA ( b ), 100 pM of the DNA target ( c ), large excess (1 μM) of a three-base mismatched oligonucleotide ( d ), 10 nM two-base mismatched oligonucleotide ( e ), 10 nM target DNA ( f ), 16S rRNA corresponding to 5×10 5 CFU μl −1 E. coli ( g ) and 16S rRNA corresponding to 7×10 5 CFU μl −1 K. pneumoniae ( h ). Scale bar, 10 μm. The corresponding column graph was shown in i . Error bars estimated as a triple of the standard deviation ( n =20). *Indicates a significance value of P <0.001. Full size image The specificity of the motion-driven bioassay was also tested using a biological control, Klebsiella pneumoniae , another Gram-negative pathogenic Enterobacteriaceae [23] . As illustrated in Figure 4g, h , and contrary to the signal of E. coli 16S rRNA (average speed of 28.2 μm s −1 , Fig. 4g ), the nanomotor response to the presence of K. pneumoniae 16S rRNA (average speed of 9.7 μm s −1 , Fig. 4h ) is similar to that observed for the negative control (without target, average speed of 9.2 μm s −1 , Fig. 4a ). This shows the high specificity of the motion bioassay towards the E. coli 16S rRNA target (versus other non-complementary bacterial RNAs) and to the absence of non-specific adsorption of SH-DP-Ag NPs. These results show the high specificity of the selected capture probe for binding only 16S rRNA in E. coli lysates, despite the potential conservation of the 16S rRNA gene. The precision of the new motion-driven biodetection platform was also examined. Supplementary Figure S4a shows speed signals of ten different nanomotors for a 1 nM DNA target solution. Well-defined and reproducible speed signals are observed, leading to a favourable relative standard deviation of 5.66%. Similarly, nanomotor speed variability between three different experimental batches revealed negligible differences ( P <0.05) in connection with the 1 nM DNA target, as shown in Supplementary Figure S4b . We have shown the first example of practical realization of synthetic nanomotors as a bioanalytical tool, in connection with the detection of DNA and bacterial rRNA. Such motion-based DNA sensing relies on the use of an optical microscope for directly tracking changes in the speed of unmodified nanowire motors. The silver-ion-induced nanomotor acceleration reflects the sandwich formation among the capture probe, complementary target and the SH-DP-Ag NPs. The nanoparticle-induced nanomotor acceleration reflects the dramatically enhanced speed of catalytic nanomotors in the presence of silver ion. The resulting motion-driven biodetection strategy offers sensitive and selective, easily measured distance readouts down to the 40 amol DNA level and the ability to directly detect raw bacterial ribosomal RNA without isolation or purification steps. Unlike common nanoparticle-based silver enhancement DNA optical [17] or electrochemical [18] hybridization assays, the nanomotor method requires no such particle enlargement (and hence is not susceptible to non-specific Ag precipitation) and relies on portable, simple and low-cost instrumentation. Motion-based biosensing can be expanded to multiplexed measurements of multiple targets by encoding functionalized nanomotors with a multi-stripe barcode segment. The template nanowire preparation route allows adding a multi-stripe Ag–Au section to the Au–Pt nanomotor, thus facilitating rapid reflectivity identification. An internal standard could also be used in the new motion detection to facilitate the quantitation of the nucleic acid target and address rare potential variations between nanomotor batches. It is also worth noting that the new nanomotor speed transduction facilitates the collection of multiple readings in a single experiment, thereby contributing to the overall reliability of the proposed protocol. The sensitivity and selectivity could be even further enhanced by recording the distance signals over longer periods of time and by using specific peptide nucleic acid probes, respectively. As the sensitivity of real-life nucleic acid measurements is commonly limited by non-specific adsorption signals, we used here a new multi-component ternary monolayer that effectively minimizes such non-specific background contributions compared with commonly used binary monolayers. A huge excess of non-complementary DNA or rRNA from a different bacteria thus has a negligible effect on the fully complementary target (DNA or rRNA) distance signals. Motion-driven biosensing represents a new paradigm in bioanalysis, as it relies for the first time on speed and distance as the analytical signals. Although the concept has been presented in connection with motion-based DNA biodetection and Ag NP tags, it may be extended to the detection of a broad range of target biomolecules in connection with different biomolecular interactions and motion transduction principles. Such new approaches to transduce the biomolecular recognition event into nanomotor motion are currently being examined in our laboratory. The distance signals can be translated into analytical results using low-cost microscopic readers, thereby making the new method affordable and attractive for low-resource settings. Owing to its attractive features, we expect that the new motion-based signal transduction will lead to a host of new and powerful biosensing applications, including clinical diagnostics, biothreat detection, food safety and forensic analysis. Reagents Silver nanoparticles (diameter 20±5 nm given by the manufacturer) were purchased from Ted Pella (cat no. 15705-20SC). MCH, sodium dodecyl sulphate (SDS), DTT, trizma hydrochloride (Tris-HCl), ethylenediaminetetraacetic acid and bovine serum albumin were obtained from Sigma-Aldrich and used without further purification. The blocking agent casein was obtained from Pierce. The buffer solutions used were as follows: The DNA immobilization buffer was 10 mM Tris-HCl, 1 mM ethylenediaminetetraacetic acid and 0.3 M NaCl (pH 8.0). The hybridization buffer (HB) was a 1 M phosphate buffer solution containing 2.5% bovine serum albumin and 0.05% casein (pH 7.2). The storage buffer for SH-DP-Ag NPs contained 10 mM phosphate buffer, 300 mM NaCl and 0.01% SDS (pH 7.2). The sequences of the oligomers used for the detection of synthetic 30-mer oligonucleotides or E. coli 16S rRNA targets are given in the Supplementary Table . All thiolated oligonucleotides were purchased from Integrated DNA Technologies. Other oligonucleotides, that is, the complementary and non-complementary targets, were obtained from Thermo Fisher Scientific. According to the sandwich protocol, SH-CP was immobilized on the gold surface, whereas SH-DP was conjugated with Ag nanoparticle tags. Bacterial strains of E. coli (NEB 5-α) and K. pneumoniae (KP210) were obtained from the University of California, Los Angeles. The isolates were stored at −80 °C and were freshly lysed before each experiment. Preparation of nanomotors The Au–Pt nanomotors were prepared by sequential electrodeposition of gold and platinum into 200-nm-diameter nanopores of a 60-μm-thick alumina membrane template (cat. no. 6809-6022, Whatman) [13] . Briefly, the branched side of the membrane was sputtered with a thin gold film, followed by electrodeposition of a sacrificial copper layer from a 1 M cupric sulphate pentahydrate solution (CuSO 4 .5H 2 O, Sigma-Aldrich), using a charge of 10 C and a potential of −1.0 V (versus Ag/AgCl reference electrode), along with a platinum wire counter electrode. Subsequently, the Au segment was plated from a gold plating solution (Orotemp 24 RTU RACK; Technic) and electrodeposited at a total charge of 1.5 C and a potential of −0.9 V. Platinum was then deposited galvanostatically using a current of −2 mA for 50 min from a platinum plating solution (Platinum RTP; Technic). Similarly, magnetic Au–Ni–Au–Pt nanomotors were prepared by introducing a ferromagnetic Ni segment. Following an initial deposition of gold segment at 0.75 C, Ni was electrodeposited at −1.0 V for 2 C (versus Ag/AgCl) from a plating solution (20 g l −1 NiCl 2 6H 2 O, 515 g l −1 Ni(H 2 NSO 3 ) 2 4H 2 O and 20 g l −1 H 3 BO 3 (buffered to pH 3.4)). Subsequently, the second gold segment (0.75 C) and a platinum segment were electrodeposited as above. The sputtered gold layer and the copper sacrificial layer were sequentially removed by mechanical polishing using cotton tip applicators soaked with 0.5 M CuCl 2 solution in 20% HCl. The nanomotors were then released by immersing the membrane in 3 M NaOH for 30 min. The synthesized nanomotors were separated from solution by centrifugation at 2,300 g for 5 min and washed repeatedly with ultrapure water (18.2 MΩ cm) until a neutral pH was achieved. Between the washing steps, the nanomotor suspension was mixed with ultrapure water and briefly sonicated to ensure the complete dispersion of nanomotors. All nanomotors were stored in ultrapure water at room temperature and their speed was tested before each experiment to identify potential nanomotor 'malfunction'. Conjugation of SH-DP with Ag NPs The SH-DP-Ag NPs were prepared in accordance with earlier studies [24] , [25] , [26] , [27] . The silver colloid (0.12 nM given by the manufacturer) was concentrated ten times by centrifugation (16,770 g , 15 min) and redispersed in nanopure water to yield a final concentration of 1.2 nM. Appropriate aliquots of SH-DP were added (final concentration 10 μM) to 100 μl of the 1.2 nM Ag NPs solution and incubated for 2 h. The SDS solution (1%) and 100 mM (pH 7.2) phosphate buffer solution were added to the above mixture to reach final concentrations of 0.01% and 10 mM, respectively. The solution was kept for gentle shaking overnight. Small aliquots of 2 M NaCl were added over 48 h to raise the final NaCl concentration to 500 mM, followed by another overnight incubation. Subsequently, the excess of SH-DP was removed by centrifugation (24,150 g , 10 min) and redispersed in storage buffer, a procedure repeated three times. Assembling the capture probe at the gold surface DNA hybridization was performed on an array of 16 gold electrodes (each 2.5 mm diameter; GeneFluidics.). Initially, 10 μM of freshly prepared DTT was added to SH-CP (0.5 μM) in immobilization buffer and allowed to stand for 10 min. A 6 μl aliquot of this SH-CP solution was drop cast to cover each Au sensor and stored overnight at 4 °C in a humidified environment. After washing with ultrapure water, the probe-modified Au sensors were treated with 6 μl of the 1 mM MCH aqueous solution for 50 min to obtain a ternary self-assembled monolayer. Finally, the sensors were thoroughly rinsed with ultrapure water and dried under nitrogen. DNA hybridization assay The DNA detection strategy is illustrated in Figure 1 . Different concentrations of the DNA target (or non-complementary and mismatched oligos) were prepared in HB. Aliquots (4 μl) of this target solution were cast on each SH-CP-modified gold sensor and incubated for 15 min. After the sensors were slightly rinsed by ultrapure water and dried by N 2 , a 4 μl of SH-DP-Ag NPs conjugation solution was cast on each sensor and was incubated for 30 min. After incubation, each sensor was thoroughly rinsed and subsequently washed with ultrapure water in a shaker (300 r.p.m.) for 5 min and dried with N 2 . These sensors were immediately used for the nanomotor-based hybridization assay. Bacterial 16S rRNA hybridization assay The bacterial 16S rRNA target, derived from single-step bacterial lysis [20] , was detected using the same SH-CP and Ag NPs-modified detector probe, in a manner similar to the synthetic 30-mer target DNA detection. The bacteria were initially lysed by resuspending the appropriate pellet containing ∼ 10 7 CFU bacteria in 10 μl of 1 M NaOH and incubating for 5 min. A 50 μl aliquot of HB was added to this 10 μl bacterial lysate, leading to genetic material corresponding to ∼ 10 7 CFU per 60 μl (final pH 7.8). This solution was serially diluted in HB to provide different concentrations of bacterial genetic material (16S rRNA). Aliquots (4 μl) of this raw bacterial target were cast on each capture probe-modified sensor for 15 min, followed by hybridization with SH-DP-Ag NPs, and washing, dissolution and detection steps. All procedures were carried out at room temperature. Nanomotor motion-based readout for hybridization detection Silver-ion-induced motion-based sensing protocol described earlier [13] was used for detecting DNA and E. coli 16S rRNA. For this purpose, 5 μl of H 2 O 2 (30%) was dropped on the sensor modified with the sandwich-hybridized duplexes for 2 min to dissolve Ag NPs to Ag + . The assay was completed by mixing the above Ag + -enriched H 2 O 2 fuel solution with equal volume of freshly prepared nanomotors in ultrapure water. The resulting mixed solution was then added to the glass slide for immediate video acquisition and tracking. Nanomotors were tracked following the protocol reported earlier [13] , [28] . An inverted optical microscope (Nikon Instrument, Eclipse TE2000-S) equipped with a 40× objective, a Photometrics CoolSnap CF camera (Roper Scientific) and MetaMorph 7.1.7 software (Molecular Devices) was used for capturing movies at a frame rate of 10 fps. This software calculates the instantaneous velocity by tracking the object's center-to-center displacement from frame to frame. Usually, five videos from randomly selected glass slide areas (200 μm×200 μm) were recorded to ensure accurate population sampling. Approximately, 20 random nanomotors were tracked for 50 frames to obtain a representative nanomotor speed. Bonferroni-corrected analyses of variance (ANOVAs) ( P <0.05) and power calculations were performed on all data sets to determine the detection limit and identify statistically significant concentrations. How to cite this article: Wu, J. et al . Motion-based DNA detection using catalytic nanomotors. Nat. Commun. 1:36 doi: 10.1038/ncomms1035 (2010).